A sex-specific transcription factor controls male identity in a simultaneous hermaphrodite Evolutionary transitions between hermaphroditic and dioecious reproductive states are found in many groups of animals. To understand such transitions, it is important to characterize diverse modes of sex determination utilized by metazoans. Currently, little is known about how simultaneous hermaphrodites specify and maintain male and female organs in a single individual. Here we show that a sex-specific gene, Smed-dmd-1 encoding a predicted doublesex/male-abnormal-3 (DM) domain transcription factor, is required for specification of male germ cells in a simultaneous hermaphrodite, the planarian Schmidtea mediterranea . dmd-1 has a male-specific role in the maintenance and regeneration of the testes and male accessory reproductive organs. In addition, a homologue of dmd-1 exhibits male-specific expression in Schistosoma mansoni , a derived, dioecious flatworm. These results demonstrate conservation of the role of DM domain genes in sexual development in lophotrochozoans and suggest one means by which modulation of sex-specific pathways can drive the transition from hermaphroditism to dioecy. Evolutionary transitions between hermaphroditic and dioecious reproductive states are found in many different groups of animals [1] , [2] , [3] . To understand such transitions, it is important to characterize diverse modes of sex determination and differentiation utilized by sexually reproducing metazoans. Previous studies have described the genetic and/or environmental factors that determine male or female identity in developing embryos of dioecious organisms [4] , [5] , [6] . Following sex determination, a cascade of mechanisms promotes the differentiation of sexual organs and enables germ cells to adopt their sexual identity [7] , [8] . The sexual fate of germ cells in dioecious organisms may be influenced solely by the sex of the somatic environment [9] , [10] , or by a combination of cues from both the soma and germ cells [11] , [12] , [13] . In contrast to dioecious organisms, simultaneous hermaphrodites produce gametes and accessory reproductive organs of both sexes. In spite of all that has been learned about sex determination mechanisms in dioecious animals, little is known about how simultaneous hermaphrodites with no sex chromosomes specify and maintain the fates of male and female germ cells as well as sexually dimorphic somatic structures in the same body. In many dioecious species, doublesex/male-abnormal-3 (DM) domain genes have critical roles in sex-specific development and function [14] , [15] , [16] , [17] , [18] , [19] , [20] , [21] . To examine whether such sex-specific functions may also function in simultaneous hermaphrodites, we investigated the role of DM domain genes in the planarian, Schmidtea mediterranea . Here, we show that proper development of the hermaphroditic reproductive system in the planarian S. mediterranea is regulated by a gene encoding a DM domain transcription factor, Smed-dmd-1 . dmd-1 messenger RNA (mRNA) is expressed in somatic cells associated with the testes and in male, but not female, accessory reproductive organs. Abrogation of dmd-1 function results in defects in germline specification and the initial differentiation of the reproductive system. In addition, dmd-1 has a male-specific role in the maintenance and regeneration of the testes and male accessory reproductive organs. These results demonstrate that dmd-1 is an essential component of pathways responsible for inductive specification of the germline and development of a sex-specific somatic gonadal niche in a simultaneous hermaphrodite. We also show that a homologue of dmd-1 exhibits sex-specific expression in S. mansoni , a derived, dioecious flatworm, suggesting a means by which modulation of sex-specific pathways may drive the transition from hermaphroditism to dioecy. Furthermore, our study of dmd-1 in two flatworm species provides evidence for the conservation of sex regulatory function between lophotrochozoans and other metazoans. Identification of Smed-dmd-1 We identified four genes containing conserved DM domains in the genome of S. mediterranea ( Supplementary Table S1 ). Sequence comparisons using BLAST (ref. 22 ) of the predicted DM domain protein sequences did not detect significant sequence similarities to other DM domain proteins outside the DM domain, consistent with previous phylogenetic analysis of DM domain genes [23] . A maximum likelihood analysis using only the DM domains from each gene was used to generate a phylogenetic tree. Although the tree had poor resolution, and low bootstrap support across most of the topology, it provided evidence of moderate-to-strong relationships between Smed-dmd-1 and homologues in S. mansoni ( Sm_dmd-1 and Sm_dmd-2 , GenBank/EMBL/DDBJ accession numbers XM002575184.1 and XM002574366.1 ) and the liver fluke, Clonorchis sinensis ( dmrt-1a and dmrt-1b , GenBank/EMBL/DDBJ accession numbers GAA52246.1 and GAA34150.2 ) ( Supplementary Fig. S1 ). By contrast, dmd-2, -3 and - 4 of S. mediterranea do not have obvious close homologues in other species based on phylogenetic reconstructions using DM domain or BLAST comparisons using the full protein sequence. Expression of dmd-1 in sexual and asexual planarians We used whole-mount in situ hybridization (WISH) to investigate the expression of the four DM domain genes in the planarian, S. mediterranea. Of the four genes, only Smed-dmd-1 mRNA transcripts were detected in the reproductive system. We cloned four splice variants of dmd-1 , with the longest open reading frame encoding a predicted protein of 341 aa ( Supplementary Table S1 , Supplementary Fig. S2 ). An individual planarian’s reproductive system consists of both male and female gonads, as well as accessory reproductive organs (for example, oviducts, sperm ducts and seminal vesicles) [24] . In these hermaphrodites, the male gonads are located dorsolaterally and the female gonads are located ventrally at the base of the brain. Germline stem cells associated with the testes and ovaries can be identified by expression of the germline-specific marker, nanos [24] , [25] , [26] , [27] (GenBank/EMBL/DDBJ accession number EF035555.1 , Fig. 1a ). Notably, asexual strains of planarians that reproduce strictly by transverse fission also contain nanos -positive germ cells, but these cells fail to differentiate [24] , [25] , [26] , [27] . In mature sexual animals, dmd-1 transcripts were detected by WISH in a subset of cells within and in close proximity to the testes ( Fig. 1b ), in the brain (br, Fig. 1c ), and in male accessory reproductive organs (seminal vesicles, sv; sperm ducts, sd; and penis papilla, pp; Fig. 1c ). Using two-colour fluorescent in situ hybridization (FISH), we found that the dorsolateral dmd-1 -expressing cells reside in close proximity to the testes primordia in recently hatched animals ( Fig. 1d ), and are found in the developing testes in sexually immature planarians ( Fig. 1e ). Similarly, in the asexual strain, we detected dmd-1 -expressing cells in the germ cell clusters along the dorsolateral region of the animal ( Fig. 1f ), the location of the presumptive testes. We also used transmission electron microscopy (TEM) to visualize the dorsolateral germ cell clusters in asexual planarians. Within these germ cell clusters, we found somatic cells with processes surrounding the germ cells. Somatic and germ cells were distinguishable owing to marked differences in the electron density of their cytoplasm and peripheral condensations of heterochromatin in the somatic cells ( Fig. 1g ). The somatic cells seen by TEM likely correspond to dmd-1 -expressing cells. Consistent with this idea, the dmd-1 -positive cells in the testes of mature sexual planarians did not express germ cell markers, including nanos [25] , [26] , [27] , germinal histone H4 (ref. 27 ) (GenBank/EMBL/DDBJ accession number DN306099 ) and msy4 (refs 28 , 29 ) (GenBank/EMBL/DDBJ accession number BK007100.1 ) ( Fig. 1h–j ), suggesting that these are somatic cells of the testes. 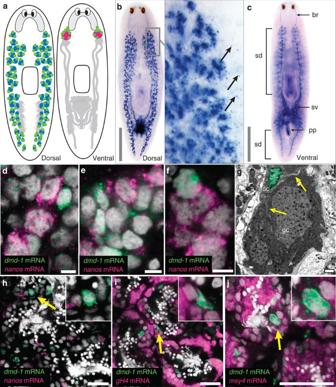Figure 1:dmd-1is expressed in the somatic cells of the male reproductive system. (a) Generalized reproductive system in the sexual planarian. Left, testes (blue) are located dorsolaterally. Right, ovaries (pink) are located more ventrally at base of the brain.nanos-positive germline stem cells of the testes and ovaries (green). Accessory reproductive structures (grey). (b) WISH showingdmd-1transcripts in and around (arrows) the testes in a sexually mature planarian. (c) Ventral view of the animal showingdmd-1transcripts in the brain (br), sperm ducts (sd), seminal vesicles (sv) and penis papilla (pp) of a sexually mature planarian. (d–f) Single confocal sections showing two-colour FISH fordmd-1(green) andnanos(magenta) mRNAs in the testes primordia of animals <24 h after hatching (d), developing testes of sexually immature planarians (e) and germ cell clusters in asexuals (f). (g) TEM showing germ (gc) and somatic cells (sc, nucleus pseudo-coloured green, arrows indicate processes) in an asexual planarian. (h–j) Single confocal sections showing two-colour FISH fordmd-1(green) and germ cell markers (magenta). Somatic cells expressingdmd-1in the testes do not express germ cell markersnanos(h, 124/125 cells aredmd-1+/nanos−),gH4(i, 136/136 cells aredmd-1+/gH4−) andmsy4(j,129/129 cells aredmd-1+/msy4+). Cell counts were performed from 25–38 testes lobes in at least two animals. Insets, magnified views show cells expressingdmd-1transcripts (yellow arrows). Scale bars:b,c, 1,000 μm;d–f, 5 μm;g, 1 μm;h–j, 25 μm. Figure 1: dmd-1 is expressed in the somatic cells of the male reproductive system. ( a ) Generalized reproductive system in the sexual planarian. Left, testes (blue) are located dorsolaterally. Right, ovaries (pink) are located more ventrally at base of the brain. nanos -positive germline stem cells of the testes and ovaries (green). Accessory reproductive structures (grey). ( b ) WISH showing dmd-1 transcripts in and around (arrows) the testes in a sexually mature planarian. ( c ) Ventral view of the animal showing dmd-1 transcripts in the brain (br), sperm ducts (sd), seminal vesicles (sv) and penis papilla (pp) of a sexually mature planarian. ( d – f ) Single confocal sections showing two-colour FISH for dmd-1 (green) and nanos (magenta) mRNAs in the testes primordia of animals <24 h after hatching ( d ), developing testes of sexually immature planarians ( e ) and germ cell clusters in asexuals ( f ). ( g ) TEM showing germ (gc) and somatic cells (sc, nucleus pseudo-coloured green, arrows indicate processes) in an asexual planarian. ( h – j ) Single confocal sections showing two-colour FISH for dmd-1 (green) and germ cell markers (magenta). Somatic cells expressing dmd-1 in the testes do not express germ cell markers nanos ( h , 124/125 cells are dmd-1+/nanos− ), gH4 ( i , 136/136 cells are dmd-1+/gH4− ) and msy4 ( j , 129 /129 cells are dmd-1+/msy4+ ). Cell counts were performed from 25–38 testes lobes in at least two animals. Insets, magnified views show cells expressing dmd-1 transcripts (yellow arrows). Scale bars: b , c , 1,000 μm; d – f , 5 μm; g , 1 μm; h – j , 25 μm. Full size image To characterize the expression of dmd-1 in the brain, we performed two-colour FISH to visualize the neurons and dmd -1-positive cells. A subset of dmd-1 -positive cells in the brain co-expresses chat transcripts, a marker of cholinergic neurons [30] , [31] , suggesting that the dmd -1-expressing cells in the brain are neurons ( Fig. 2a ). These dmd-1 -positive neurons are detectable in animals <24 h after hatching ( Fig. 2b ), in asexual animals ( Fig. 2c ) and also in planarians regenerating new brains ( Fig. 2d , Supplementary Fig. S3 for scheme). 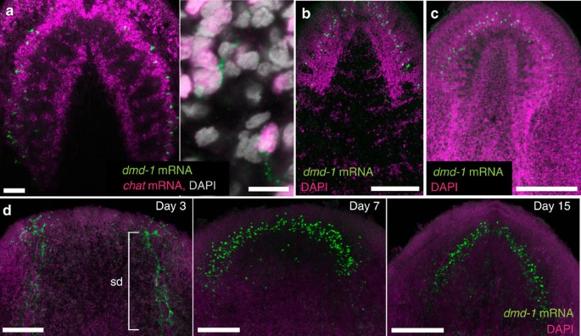Figure 2:dmd-1is expressed in some neurons in the planarian brain. (a) Left, two-colour FISH ofdmd-1andchattranscripts in the brain of a sexual planarian. Right, single confocal section showing cells co-expressingdmd-1mRNA (green) andchattranscripts (magenta), a marker of cholinergic neurons. (b)dmd-1transcripts, detected by FISH, in the brain of animals <24 h after hatching. (c)dmd-1transcripts, detected by FISH, in the brain of an asexual planarian. (d) FISH to detectdmd-1transcripts in animals during brain regeneration. The sperm ducts (sd) in the old tissue are still present in day 3 regenerates, but are barely visible owing to regression in day 7 and day 15 regenerates. (a–d) Images shown are confocal projections. Scale bars:a, 50 μm;b–d, 200 μm. Figure 2: dmd-1 is expressed in some neurons in the planarian brain. ( a ) Left, two-colour FISH of dmd-1 and chat transcripts in the brain of a sexual planarian. Right, single confocal section showing cells co-expressing dmd-1 mRNA (green) and chat transcripts (magenta), a marker of cholinergic neurons. ( b ) dmd-1 transcripts, detected by FISH, in the brain of animals <24 h after hatching. ( c ) dmd-1 transcripts, detected by FISH, in the brain of an asexual planarian. ( d ) FISH to detect dmd-1 transcripts in animals during brain regeneration. The sperm ducts (sd) in the old tissue are still present in day 3 regenerates, but are barely visible owing to regression in day 7 and day 15 regenerates. ( a – d ) Images shown are confocal projections. Scale bars: a , 50 μm; b – d , 200 μm. Full size image Expression of dmd-1 in regenerating planarians To examine the expression pattern of dmd-1 during the regeneration process, sexual planarians were amputated in the region between the ovaries and pharynx ( Supplementary Fig. S4a ). We performed two-colour FISH at several time points to detect dmd-1 and gH4 (to aid in visualization of neoblasts and germ cells) transcripts. At 3 days post amputation, we detected dmd-1 -positive cells in and around the testes lobes in the old tissue, and in the early blastema of the regenerating anterior fragment ( Supplementary Fig. S4b ). Between 7 and 10 days post amputation, dmd-1 -positive cells were present in the blastema, as well as in and around the regressed testes lobes in the old tissue ( Supplementary Fig. S4c ). At 15 days post amputation, dmd-1 -positive cells were detected within the new testes lobes that formed in the newly regenerated posterior end of the animal ( Supplementary Fig. S4d , right panel, top). We also observed a cluster of dmd-1 -expressing cells just posterior to the pharynx where the copulatory apparatus is located in sexually mature animals, suggesting that such cells may develop into the male accessory reproductive organs ( Supplementary Fig. S4d , left and right panels, yellow box). dmd-1 is expressed in differentiating neoblast progeny In addition to the dmd-1 -positive somatic cells in the testes, dmd-1 -positive cells are found in close proximity to the testes lobes in the dorsolateral region. In planarians, pluripotent stem cells (cNeoblasts) provide new cells for regeneration and physiological cell turnover in the animal [32] . Neoblasts are irradiation-sensitive and are depleted within 24 h following irradiation, while their differentiating progeny are lost with different kinetics, becoming depleted several days after irradiation [33] . Neoblasts express abundant smedwi-1 mRNA (GenBank/EMBL/DDBJ accession number DQ186985.1 ), whereas SMEDWI-1 protein is detected in neoblasts and their differentiating progeny [34] , [35] . By combined FISH and immunostaining, we detected smedwi-1 mRNA and SMEDWI-1 protein in the dmd-1 -positive cells in close proximity to the testes, suggesting that they could be differentiating neoblast progeny ( Fig. 3a ). To test this idea, we irradiated asexual planarians at 100 Gy and performed quantitative real-time PCR (qPCR) to assay for dmd-1 transcripts. By 48 h post irradiation, the radiation-sensitive neoblasts and germ cells were depleted, as indicated by a dramatic decrease in smedwi-1 and nanos transcript levels compared with unirradiated controls ( Fig. 3b ). By contrast, dmd-1 transcript levels in irradiated animals decreased by ~50% relative to unirradiated controls. By day 7 post irradiation, we observed a further decrease of dmd-1 transcript levels ( Fig. 3b ). These results were confirmed by FISH: we observed a reduction of dmd-1 -positive cells at 48 h ( Fig. 3c ) and by day 7 these cells were quite rare ( Fig. 3d ). In contrast to dorsolateral dmd-1 labelling, we found no dramatic differences in the brain of irradiated versus control animals ( Fig. 3e ). Together, these data suggest that dmd-1 -positive somatic cells associated with the testes turn over within 7 days and after irradiation these somatic cells are unable to be renewed by neoblasts. 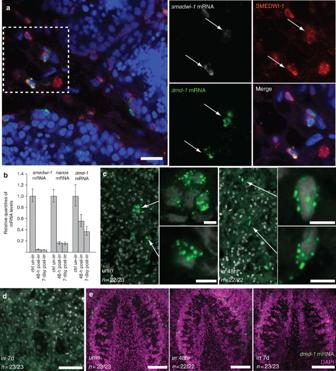Figure 3:dmd-1-positive cells in proximity to the testes are differentiating neoblast progeny. (a) Single confocal section showing two-colour FISH combined with immunostaining in mature sexual animals.dmd-1cells (green) in close proximity to the testes expresssmedwi-1transcripts (grey), a marker of neoblasts. SMEDWI-1 protein (red), a marker of neoblasts and differentiating neoblasts is also detected in thesedmd-1-positive cells. Arrows indicatedmd-1-positive cells within the dashed box. (b) qPCR showing relative levels ofsmedwi-1,nanosanddmd-1mRNAs in irradiated (100 Gy) versus unirradiated asexual planarians 48 h and 7 days post irradiation. Error bars indicate 95% confidence intervals calculated based on s.e.m., results are the mean from three independent experiments using pools of eight planarians. (c) At 48 h after irradiation,dmd-1-positive cells (arrows) are present in the dorsolateral region of the animal, albeit in fewer numbers, compared with control animals. Magnified views of cells expressingdmd-1transcripts (insets).dmd-1transcripts were detected by FISH. Images shown are single confocal sections. (d) At 7 days after irradiation,dmd-1-positive cells are rarely detectable in the dorsolateral region of the animal.dmd-1transcripts were detected by FISH. Images shown are single confocal sections. (e) Confocal projection showing thatdmd-1-positive cells (detected by FISH) are still present in the brain at 48 h and 7 days after irradiation. Scale bars:a, 20 μm;c, 5 μm;d, 50 μm;e, 100 μm. Figure 3: dmd-1 -positive cells in proximity to the testes are differentiating neoblast progeny. ( a ) Single confocal section showing two-colour FISH combined with immunostaining in mature sexual animals. dmd-1 cells (green) in close proximity to the testes express smedwi-1 transcripts (grey), a marker of neoblasts. SMEDWI-1 protein (red), a marker of neoblasts and differentiating neoblasts is also detected in these dmd-1 -positive cells. Arrows indicate dmd-1 -positive cells within the dashed box. ( b ) qPCR showing relative levels of smedwi-1 , nanos and dmd-1 mRNAs in irradiated (100 Gy) versus unirradiated asexual planarians 48 h and 7 days post irradiation. Error bars indicate 95% confidence intervals calculated based on s.e.m., results are the mean from three independent experiments using pools of eight planarians. ( c ) At 48 h after irradiation, dmd-1 -positive cells (arrows) are present in the dorsolateral region of the animal, albeit in fewer numbers, compared with control animals. Magnified views of cells expressing dmd-1 transcripts (insets). dmd-1 transcripts were detected by FISH. Images shown are single confocal sections. ( d ) At 7 days after irradiation, dmd-1 -positive cells are rarely detectable in the dorsolateral region of the animal. dmd-1 transcripts were detected by FISH. Images shown are single confocal sections. ( e ) Confocal projection showing that dmd-1 -positive cells (detected by FISH) are still present in the brain at 48 h and 7 days after irradiation. Scale bars: a , 20 μm; c , 5 μm; d , 50 μm; e , 100 μm. Full size image dmd-1 is required for male germ cell maintenance in asexuals To test for a functional relationship between dmd-1 -expressing somatic cells and nanos -positive early germ cells, we first knocked down dmd-1 in asexual planarians, because they lack differentiated germ cells and accessory reproductive organs. qPCR revealed a dramatic decrease in nanos expression in asexual dmd-1 -knockdown animals, relative to controls ( Fig. 4a ). We confirmed this result by FISH to detect the clusters of germ cells co-expressing gH4 and nanos . After dmd-1 RNA interference (RNAi), no gH4 / nanos co-expressing germ cells were detectable in the dmd-1 -knockdown animals ( Fig. 4b ). These data indicate that dmd-1 is required for the maintenance of the dorsolateral presumptive male germ cells in asexual planarians. We have been unable to assay the effect of dmd-1 knockdown on female germ cells, as under our experimental conditions we do not detect gH4 / nanos co-expressing germ cells in the ovarian region of either the control or RNAi animals. Interestingly, when nanos was knocked down in asexual planarians, the abundance of dmd-1 transcripts, as measured by qPCR, was unaffected ( Fig. 4c ). This result suggests that dmd-1 -positive somatic cells are not dependent on the presence of germ cells. 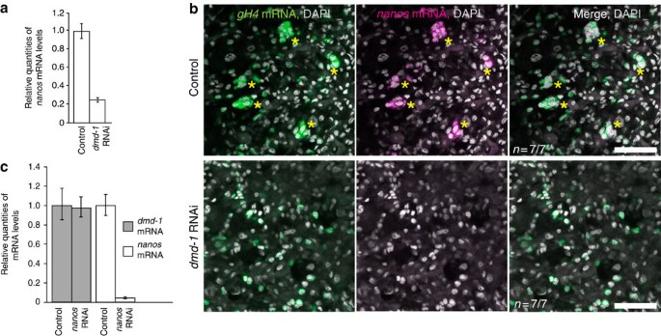Figure 4:dmd-1is required for maintenance of presumptive male germ cells in asexuals. (a) qPCR showing decreasednanostranscript levels indmd-1(RNAi) versus control asexuals. Error bars indicate 95% confidence intervals calculated based on s.e.m.,n=8 individual animals. (b) Loss ofgH4+/nanos+ germ cell clusters (asterisks) indmd-1(RNAi) asexuals.gH4+/nanos− cells indmd-1(RNAi) animals are somatic neoblasts. Images shown are single confocal optical sections;gH4andnanosmRNAs are detected by two-colour FISH. (c) qPCR showing thatdmd-1transcript levels innanos(RNAi) versus control asexuals remain unchanged. Error bars indicate 95% confidence intervals calculated based on s.e.m., results are the mean from three independent experiments using pools of nine planarians. Scale bars:b, 50 μm. Figure 4: dmd-1 is required for maintenance of presumptive male germ cells in asexuals. ( a ) qPCR showing decreased nanos transcript levels in dmd-1 (RNAi) versus control asexuals. Error bars indicate 95% confidence intervals calculated based on s.e.m., n =8 individual animals. ( b ) Loss of gH4 +/ nanos + germ cell clusters (asterisks) in dmd-1 (RNAi) asexuals. gH4 +/ nanos − cells in dmd-1 (RNAi) animals are somatic neoblasts. Images shown are single confocal optical sections; gH4 and nanos mRNAs are detected by two-colour FISH. ( c ) qPCR showing that dmd-1 transcript levels in nanos (RNAi) versus control asexuals remain unchanged. Error bars indicate 95% confidence intervals calculated based on s.e.m., results are the mean from three independent experiments using pools of nine planarians. Scale bars: b , 50 μm. Full size image dmd-1 is required to regenerate male germ cells de novo The germline of S. mediterranea can be regenerated de novo from somatic tissue [27] , implying that the planarian germline is specified inductively [24] . Both nanos and dmd-1 mRNAs are detectable in sexual animals <24 h post hatching ( Fig. 1d ), suggesting that dmd-1 may be involved in the inductive specification of the germline. To examine this possibility, we knocked down dmd-1 in sexual worms, and amputated their heads anterior to the ovaries, generating fragments devoid of reproductive tissue ( Fig. 5a ). Previous work has shown that de novo specification of the planarian germline occurs between 7–14 days post amputation [27] . Consistent with dmd-1 being required for germ cell specification, we find that a majority of dmd-1 (RNAi) animals fail to regenerate the dorsolateral clusters of nanos -positive male germ cells ( Fig. 5b ). 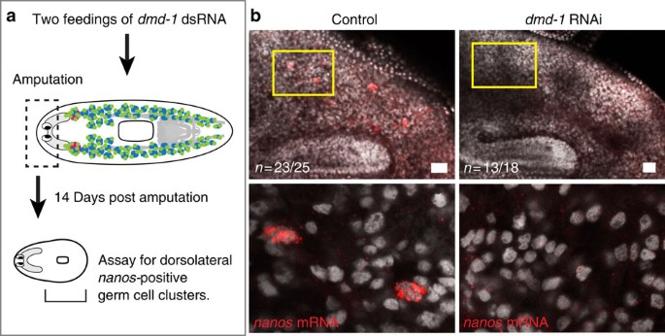Figure 5:dmd-1is required for male germ cell specification. (a) Experimental scheme for generating animals devoid of germ cells and reproductive structures. Only animals that had successfully regenerated (indicated by presence of pharynx) were scored. (b) By 14 days post amputation, planarians devoid of germ cells regenerate dorsolateralnanos-positive cells;dmd-1(RNAi) animals fail to regenerate dorsolateralnanos-positive cells. Images shown are single confocal sections;nanostranscripts are detected by FISH. Scale bars:b, 50 μm. Figure 5: dmd-1 is required for male germ cell specification. ( a ) Experimental scheme for generating animals devoid of germ cells and reproductive structures. Only animals that had successfully regenerated (indicated by presence of pharynx) were scored. ( b ) By 14 days post amputation, planarians devoid of germ cells regenerate dorsolateral nanos -positive cells; dmd-1 (RNAi) animals fail to regenerate dorsolateral nanos -positive cells. Images shown are single confocal sections; nanos transcripts are detected by FISH. Scale bars: b , 50 μm. Full size image dmd-1 is required for the initial development of germ cells To investigate the role of dmd-1 in post-embryonic development of the germline, we initiated dmd-1 RNAi in recently hatched planarians (<2 weeks old). At this early stage, nanos -positive germline stem cells are present in the gonadal primordia but the accessory reproductive organs have not yet developed. When the animals reached maturity, we found that the testes ( Fig. 6a ) and ovaries ( Fig. 6c ) were absent in dmd-1 (RNAi) animals. These results suggest that dmd-1 is required for the initial development of both male and female reproductive systems. 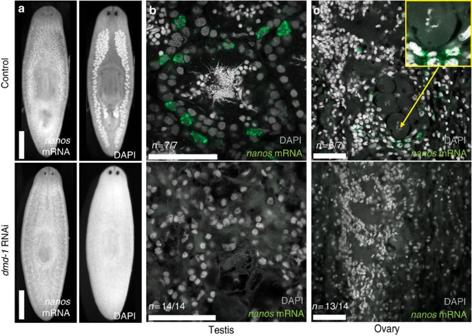Figure 6:dmd-1is required for the initial development of the reproductive system. (a) Whole-mount images showingnanostranscripts (detected by FISH) present in control but notdmd-1(RNAi) animals. The testes lobes are visible by 4',6-diamidino-2-phenylindole (DAPI) staining in the control but notdmd-1(RNAi) animals. (b) The testes are absent andnanos-positive germline stem cells are not detected indmd-1(RNAi) animals. (c) The ovaries are absent andnanos-positive germline stem cells are not detected indmd-1(RNAi) animals. Inset, magnified view of oocyte. (b,c) Images shown are single confocal sections,nanostranscripts are detected by FISH. Scale bars:a, 1 mm;b,c, 50 μm. Figure 6: dmd-1 is required for the initial development of the reproductive system. ( a ) Whole-mount images showing nanos transcripts (detected by FISH) present in control but not dmd -1(RNAi) animals. The testes lobes are visible by 4',6-diamidino-2-phenylindole (DAPI) staining in the control but not dmd -1(RNAi) animals. ( b ) The testes are absent and nanos -positive germline stem cells are not detected in dmd -1(RNAi) animals. ( c ) The ovaries are absent and nanos -positive germline stem cells are not detected in dmd -1(RNAi) animals. Inset, magnified view of oocyte. ( b , c ) Images shown are single confocal sections, nanos transcripts are detected by FISH. Scale bars: a , 1 mm; b , c , 50 μm. Full size image dmd-1 is required to maintain male germ cells in sexuals Next, we examined the role of dmd-1 in germ cell maintenance by knocking down dmd-1 in sexually mature planarians with fully developed gonads and accessory reproductive organs. In contrast to the previous experiments on hatchlings, only the male reproductive system was affected. The dmd-1 (RNAi) animals lost their testes but showed no observable defects in the ovaries ( Fig. 7a ). These observations indicate that dmd-1 is required for the maintenance of the male, but not the female, gonads in S. mediterranea . 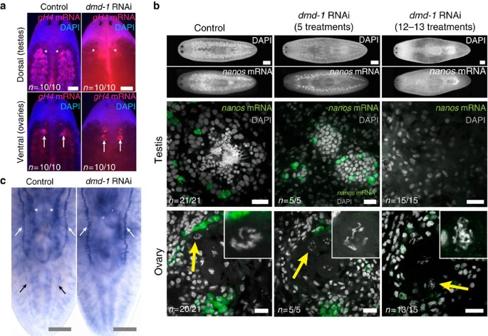Figure 7:dmd-1is required for differentiation and maintenance of male germ cells. (a) FISH was performed to detectgH4transcripts in the testes and ovaries of control anddmd-1(RNAi) animals. Whole-mount images show the loss of testes in knockdown but not control animals; the ovaries are unaffected by the knockdown. (b) The testes and ovaries of control anddmd-1(RNAi) animals visualized by 4',6-diamidino-2-phenylindole (DAPI) and FISH to detectnanostranscripts. Top panels, whole-mount images showing the testes of control and knockdown animals after 5 or 12–13 RNAi treatments. Centre panels, single confocal sections showingdmd-1(RNAi) animals lacking differentiated germ cells in the testes (5 treatments, 1 month) or devoid of testes entirely (12–13 treatments, 3 months). Bottom panels, single confocal sections showing ovaries with normal oocyte formation (arrow, inset) in control and knockdown animals. (c) Sperm ducts (black arrows) and seminal vesicles (asterisks) are absent afterdmd-1RNAi, oviducts are unaffected (n=0/5 had sperm ducts/seminal vesicles, compared with 5/5 in controls;n=4/5 had oviducts, compared with 5/5 in controls). These components of the male and female reproductive system were visualized by WISH to detecteyes absenttranscripts. Scale bars μm:a,b(whole-mounts),c, 500 μm;b, 20 μm. Figure 7: dmd-1 is required for differentiation and maintenance of male germ cells. ( a ) FISH was performed to detect gH4 transcripts in the testes and ovaries of control and dmd-1 (RNAi) animals. Whole-mount images show the loss of testes in knockdown but not control animals; the ovaries are unaffected by the knockdown. ( b ) The testes and ovaries of control and dmd-1 (RNAi) animals visualized by 4',6-diamidino-2-phenylindole (DAPI) and FISH to detect nanos transcripts. Top panels, whole-mount images showing the testes of control and knockdown animals after 5 or 12–13 RNAi treatments. Centre panels, single confocal sections showing dmd-1 (RNAi) animals lacking differentiated germ cells in the testes (5 treatments, 1 month) or devoid of testes entirely (12–13 treatments, 3 months). Bottom panels, single confocal sections showing ovaries with normal oocyte formation (arrow, inset) in control and knockdown animals. ( c ) Sperm ducts (black arrows) and seminal vesicles (asterisks) are absent after dmd-1 RNAi, oviducts are unaffected ( n =0/5 had sperm ducts/seminal vesicles, compared with 5/5 in controls; n =4/5 had oviducts, compared with 5/5 in controls). These components of the male and female reproductive system were visualized by WISH to detect eyes absent transcripts. Scale bars μm: a , b (whole-mounts), c , 500 μm; b , 20 μm. Full size image dmd-1 is required to regenerate male reproductive organs Seeing the difference in phenotype between dmd-1 knockdown in hatchlings versus sexually mature planarians, we also examined the function of dmd-1 in animals that were regenerating their reproductive system (sexually immature regenerates, Supplementary Fig. S5 ). After 1 month of dmd-1 knockdown, most testes lobules in treated animals lacked spermatids and mature sperm. Animals treated for 3 months lost their testes entirely, including the nanos -positive germ cells. Ovaries, however, were normal in both control and dmd-1 -knockdown animals, exhibiting nanos -positive germ cells and normal oocyte formation by 4',6-diamidino-2-phenylindole staining ( Fig. 7b ). These results suggest that dmd-1 is required for the differentiation of male germ cells during regeneration of the reproductive system. We also examined the effect of dmd-1 knockdown on accessory organs associated with the male and female reproductive systems. Consistent with our observations on the male germline, knockdown of dmd-1 in sexually immature regenerates resulted in the absence of sperm ducts ( Fig. 7c , black arrows) and seminal vesicles ( Fig. 7c , asterisks), as visualized by ISH with eyes absent [36] (GenBank/EMBL/DDBJ accession number EG345430.1 ), a marker for oviducts, sperm ducts and seminal vesicles ( Fig. 7c ). Again, female structures were unaffected, as we found oviducts (white arrows) in both control and knockdown animals ( Fig. 7c ). Furthermore, dmd-1 -knockdown animals still produced egg capsules ( dmd-1 RNAi: 30 egg capsules, control: 26 egg capsules; 19 animals tracked from 6th to 9th feeding over 27 days), suggesting that not only oviducts, but all female organs responsible for egg production (for example, yolk glands and cement glands— Supplementary Fig. S6 ) are functional. These findings demonstrate that dmd-1 is a component of the pathway required for the differentiation of male accessory reproductive organs. Sm_dmd-1 is expressed in male schistosomes We have shown that regeneration and maintenance of male versus female reproductive organs in a simultaneous hermaphrodite are directed by distinct molecular pathways. The presence of sex-specific pathways involved in the regeneration and maintenance of reproductive organs provides a plausible mechanism for the evolution of distinct sexes from simultaneous hermaphrodites. Though organisms within the phylum Platyhelminthes are largely hermaphroditic [37] , members of the parasitic family Schistosomatidae exist as separate male and female sexes. The dioecy of schistosomes appears to be a derived feature of this clade [1] ( Fig. 8a ). Using qPCR, we found that in S. mansoni , the homologue of dmd-1, Sm_dmd-1 is dramatically upregulated in male schistosomes, relative to females ( Fig. 8b ); thus the sex-specific expression of dmd-1 is retained in a dioecious species of the flatworm phylum. 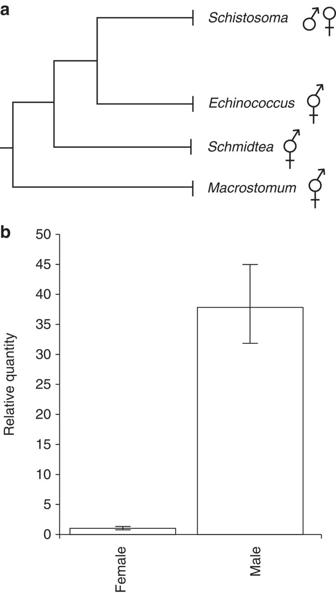Figure 8: A homologue ofdmd-1shows male-specific expression in the derived dioecious flatwormS. mansoni. (a) Simplified phylogenetic tree of the Platyhelminthes, adapted from Phylogenetic relationships of Platyhelminthes based on 18S ribosomal gene sequences60. Members of the Platyhelminthes are largely hermaphroditic (); separate male (♂) and female (♀) sexes in the schistosomes are a derived feature of this clade. (b) qPCR showing male-specific expression of admd-1homologue in the maleS. mansoni.Error bars indicate 95% confidence intervals calculated based on s.e.m., results are the mean from pools of male or female schistosomes harvested from three separate mice. Figure 8: A homologue of dmd-1 shows male-specific expression in the derived dioecious flatworm S. mansoni. ( a ) Simplified phylogenetic tree of the Platyhelminthes, adapted from Phylogenetic relationships of Platyhelminthes based on 18S ribosomal gene sequences [60] . Members of the Platyhelminthes are largely hermaphroditic (); separate male (♂) and female (♀) sexes in the schistosomes are a derived feature of this clade. ( b ) qPCR showing male-specific expression of a dmd-1 homologue in the male S. mansoni. Error bars indicate 95% confidence intervals calculated based on s.e.m., results are the mean from pools of male or female schistosomes harvested from three separate mice. Full size image The contrast between the male-specific role for dmd-1 in mature sexual worms, and its effect on both male and female systems in hatchlings is noteworthy. These different effects suggest a role for the male reproductive system in the subsequent development of the female system, consistent with the protandrous nature of sexual development in S. mediterranea . This idea is also supported by the male-specific expression of dmd-1 mRNA, which is not detected in the ovaries of sexually mature animals, sexually immature regenerates or in hatchlings. Though we cannot exclude the possibilities that dmd-1 has a direct role in the initial differentiation of ovaries or that the male-specific phenotype in mature animals results from incomplete knockdown, the lack of dmd-1 expression in cells associated with female structures suggests that its effect on early ovarian development is an indirect consequence of impaired male development. In other organisms, it has been shown that interaction between the nervous system and gonads is critical for sexual reproduction. In mammals, sexual maturation and maintenance of the gonads and reproductive structures are intimately tied to the neuroendocrine system [38] , [39] . Furthermore, sexually dimorphic neurons in Drosophila melanogaster and Caenorhabditis elegans regulate sexual behaviours [40] , [41] , [42] , [43] , [44] . In planarians, the relationship between the nervous system and reproductive system has been shown by experiments in which amputation of the brain leads to regression of the testes [27] , [45] . More recent work has demonstrated the role of neuropeptide signalling in regulating the planarian reproductive system, identifying a neuropeptide Y family member, NPY8 , that is required for the development and maintenance of reproductive organs [46] . Interestingly, dmd-1 -positive cells are detected in the planarian brain at all stages of development and regeneration, as well as in asexuals. These neurons may potentially regulate various aspects of male reproductive system development and/or sex-specific behaviours. Examining the role of the dmd-1 -positive neurons will be an important direction for future research. This work provides evidence for a conserved role of the DM domain gene family in sexual development in lophotrochozoans. To date, DM domain genes across the animal kingdom have been shown to function at different positions in the sexual development hierarchy. In the ecdysozoans C. elegans and D. melanogaster , DM domain proteins regulate the development of sexually dimorphic somatic features [6] , [17] . We have shown here that in planarians, a member of the lophotrochozoan clade, dmd-1 has a similar role—this transcription factor regulates the formation of male somatic structures like the penis papilla, sperm ducts and seminal vesicles. In addition, it is probable that dmd-1 in planarians acts cell non-autonomously to specify male germ cells and to regulate their differentiation and maintenance—roles more commonly found for DM domain proteins in vertebrates [17] , [47] . Elucidating the mechanisms by which dmd-1 functions in planarians will contribute to our understanding of how the DM domain gene family acts as a central factor in the evolution of sexual development across the metazoa. Furthermore, identifying the downstream targets of dmd-1 could help reveal the nature of the signal(s) that specify germ cells in planarians. Previous studies in nematodes have shown that transitions between different mating systems can occur via mutations that affect the sex determination pathway and the regulation of gamete physiology with few pleiotropic effects on the organism [48] , [49] . Phylogenetic analyses suggest that dmd-1 and dmd-2 in the schistosome, S. mansoni , are derived from an ancestral Platyhelminthes dmd-1 gene that duplicated in the trematode lineage after its divergence from the planarians ( Supplementary Fig. S1 ). In the case of planarians and schistosomes, the male-specific expression of dmd-1 is conserved in a simultaneous hermaphrodite and a derived, dioecious flatworm. This conservation is consistent with the idea that independently regulated sex-specific developmental pathways could serve as plausible substrates for transitions between distinct mating systems. Further characterization of deeply conserved genes like dmd-1 that have sex-specific roles in simultaneous hermaphrodites and that retain sex-specific expression in dioecious species will provide a tractable system in which to investigate the transition from hermaphroditism to dioecy. Planarian culture Asexual planarians were maintained in 1 × Montjuïc salts at 21 °C (ref. 50 ) and sexual planarians in 0.75 × Montjuïc salts at 18 °C (ref. 27 ). Animals were fed organic calf liver and starved at least 1 week before use. Cloning of DM domain genes mRNA sequences for dmd-1, 2, 3 and 4 were determined using 5′ and/or 3′ RACE (RLM-Race kit, Ambion, Austin, TX) with total RNA extracted using Trizol Reagent (Invitrogen, Carlsbad, CA). PCR products were TA cloned (Rapid DNA Ligation Kit, Roche, Mannheim, Germany) into Eam11051-digested (Thermo Scientific, Logan, UT) pJC53.2 (Addgene ID: 26536) and transformed into DH5α cells. Full-length dmd-1 complementary DNA was isolated by PCR amplification (Phusion High-Fidelity PCR Master Mix, Finnzymes, Vantaa, Finland), incubated with Taq polymerase and 10 mM dATP, TA cloned into pJC53.2 and transformed into DH5α. Identity of clones was verified by sequencing. Primer sequences are listed in Supplementary Table S2 . Phylogenetic analyses Eighty-four DM domain sequences from 74 proteins (ten had two DM domains) were obtained from the Pfam 26.0 database ( http://pfam.sanger.ac.uk ) and were aligned using CLUSTALW (ref. 51 ) ( www.genome.jp/tools/clustalw/ ). Phylogenetic reconstruction was performed using MEGA 5.05 (ref. 52 ) to perform model testing and maximum likelihood testing. Model choice was performed using the Baysian information criterion to select the optimal model for amino-acid substitutions, which was the General Reverse Transcriptase model plus Gamma distributed rate variation [53] . Evolutionary history was inferred by maximum likelihood analysis. Nodal support was estimated using 500 bootstrap replicates. An initial tree for the heuristic search (using nearest neighbour interchange) was obtained automatically from a neighbour-joining tree. A discrete Gamma distribution was used to model evolutionary rate differences among sites (five categories; +G parameter=0.9267). All ambiguous positions were removed for each sequence pair and there were a total of 55 positions in the final data set. Irradiation Asexual planarians were exposed to 100 Gy of gamma irradiation using a Gammacell 220 Excel with a cobalt-60 source (Nordion, Ottawa, ON, Canada) in 2 ml of planarian salts and processed for RNA extraction or FISH at the specified time points. RNAi analyses Truncated 3′ RACE products cloned in pJC53.2 were used as templates to generate dmd-1 double-stranded RNA (dsRNA) (sequences in Supplementary Table S1 ). Animals were fed dsRNA-containing bacteria (hatchlings, sexually immature regenerates and mature adults) or dsRNA generated by in vitro transcription (IVT) (asexuals, mature adults and animals for de novo regeneration). Animals were fed sufficient dsRNA/liver to ensure excess after the animals had eaten. To generate dsRNA by IVT, templates cloned into pJC53.2 were amplified with a modified T7 oligonucleotide (5′-GGATCCTAATACGACTCACTATAGGG-3′) and cleaned up with the DNA Clean & Concentrator kit (Zymo Research, Orange, CA, D4003) [46] . Each 20 μl IVT reaction (2 μl 10 × high yield transcription buffer (0.4 M Tris pH 8.0, 0.1 M MgCl 2 , 20 mM spermidine, 0.1 M DTT), 5 μl 25 mM rNTP (Promega, Madison, WI), 1 μl T7 polymerase, 1 μl thermostable inorganic pyrophosphatase (TIPP, 2000 U ml −1 ) (New England Biolabs, Ipwich, MA), 0.5 μl recombinant ribonuclease inhibitor (RNasin, 2500 U ml −1 ) (Promega) and 0.5–2.5 μg of PCR product) was incubated at 37 °C overnight, then treated with 1 μl of RQ1 RNase-free DNase (Fisher Scientific, Pittsburgh, PA) for 20 min at room temperature [54] . Each reaction volume was brought up to 100 μl, followed by denaturating and annealing at the following temperatures: 95 °C (3 min), 75 °C (3 min), 50 °C (3 min) and room temperature (5 min). dsRNA was cleaned up by ammonium acetate precipitation (2.5 M final concentration of ammonium acetate, plus two volumes of 100% EtOH). 0.4–1 μg dsRNA was mixed with 10 μl of 3:1 liver:water mix. Control animals were fed dsRNA synthesized from the ccdB and camR-containing insert of pJC53.2. To obtain dsRNA-containing bacteria, templates were shuttled to plasmid pPR244 using a Gateway reaction (Invitrogen) and transformed into E. coli strain HT115. dsRNA-containing bacteria was prepared by inoculating 30 ml of 2xYT with kanamycin and tetracycline with 0.5 ml of overnight culture. At OD 0.3–0.4 , cultures were induced with 0.4 M isopropylthiogalactoside for 2 h (ref. 55 ). The bacterial pellet from 1.5 ml of culture was mixed with 21 μl of 3:1 liver:water mix. Control animals were fed bacteria-containing empty pPR242 vector. Feeding schedules are provided in Supplementary Table S3 . Quantitative real-time PCR To measure relative mRNA levels, total RNA was extracted from animals 7–9 days after the final dsRNA feed and reverse transcribed. qPCR was performed on an Applied Biosystems StepOne Plus Real-Time PCR system using GoTaq qPCR Master Mix with SYBR green (Promega). Triplicates were done for all samples to account for errors in pipetting. Transcript levels were normalized to β-tubulin [GB:DN305397] (planarians) and Sm_cytochrome c oxidase I [Smp_900000, GB:AF216698.1] (schistosomes). Relative quantities were calculated using the ΔΔCt calculation in the StepOne Plus Software. Oligonucleotide primer sequences are listed in Supplementary Table S2 . Riboprobe synthesis and in situ hybridization Full-length dmd-1 in pJC53.2 was used as template to generate riboprobes for in situ hybridization (ISH). IVT reactions with T3 RNA polymerase were performed using standard approaches with either digoxigenin-12-UTP (Roche), fluorescein-12-UTP (Roche) or dinitrophenol-11-UTP (PerkinElmer, Waltham, MA). Riboprobes were synthesized for 4–5 h at 37 °C, treated with RNase-free DNase (Fisher Scientific, Pittsburgh, PA), and precipitated with ammonium acetate and ethanol. For whole-mount ISH, animals were killed with 5–10% N -acetyl-cysteine (Sigma-Aldrich, St. Louis, MO) for 8–11 min, then fixed in 4% formaldehyde in PBTx (1 × PBS+0.3% Triton X-100) for 20–30 min at room temperature [56] . The strength and times of treatment/fixation was dependent on size and condition (regenerating versus intact) of the animals. Animals were bleached in 6% H 2 O 2 in MeOH overnight [56] or in formamide/H 2 O 2 for 2–3 h (ref. 57 ). Before bleaching in H 2 O 2 in MeOH, animals were permeabilized and reduced [56] . Following bleaching, animals were treated with Proteinase K (5–10 μg ml −1 , 20 min—1 h, depending on size and condition) followed by post-fixation [56] . Riboprobe concentration for hybridization ranged from 0.1–0.3 ng μl −1 . Following post-hybridization washes and blocking, animals were incubated in either anti-digoxigenin alkaline phosphatase (1:2,000 (Roche)), anti-digoxigenin peroxidase (1:1,000 (Roche)), anti-fluorescein peroxidase (1:1,000 (Roche)) or anti-dinitrophenol peroxidase (1:100 (PerkinElmer)) overnight at 4 °C. Samples were washed and developed with Fluorescein-, Cy3- or TAMRA-Tyramide using the manufacturer’s protocol (PerkinElmer) [29] or in TSA buffer (2 M NaCl, 0.1 M Boric acid, pH 8.5) [57] . For two-colour ISH, the peroxidase after the first tyramide development was quenched with either 2% H 2 O 2 in PBTX, 1 h or 0.1% sodium azide in 1 × PBS, 30 min, followed by several washes before subsequent antibody incubation. Imaging WISH images were captured on a Leica DFC420 camera mounted on a Leica M205A stereomicroscope (Leica, Wetzlar, Germany). Samples were mounted in 80% glycerol/PBTx. Whole-mount FISH images were imaged on a Zeiss Stereo Lumar V12 (Carl Zeiss, Germany). Samples were mounted in Vectashield (Vector Laboratories, Burlingame, CA). Confocal FISH images were obtained on a Zeiss LSM 710 confocal microscope (Carl Zeiss), (Plan-Apochromat 10 × /0.45, Plan-Apochromat 20 × /0.8, C-Apochromat 40 × /1.2 W korr UV–vis-IR or Plan-Apochromat 63 × /1.4 Oil DIC objectives). Samples were mounted in Vectashield. Fluorescein, Cy3/5-TAMRA and Cy5 were excited with 488, 561 and 633 nm lasers, respectively. Images were processed (cropping and annotation; brightness and contrast adjustments to entire image) using Adobe Photoshop CS4/CS5 and/or Zen 2008/9/11. Electron microscopy Asexual worms were fixed in cold 2% formaldehyde, 2.5% glutaraldehyde in EMBuffer (70 mM sodium cacodylate, 1 mM CaCl 2 , pH 7.4), excised, fixed for four additional hours, washed twice in EMBuffer and post-fixed (1% OsO 4 , 90 min, 4 °C in dark). Animals were dehydrated (20+2% uranyl acetate, 40, 60, 80, 100% ethanol), placed in acetone, and infiltrated with epoxy-embedding resin [58] . Thin (60–90 nm) sections were collected on Formvar-coated copper slot grids (Electron Microscopy Sciences, Hatfield, PA) and stained [58] . Images were acquired with a Hitachi H-7000 STEM electron microscope in transmission mode, at an accelerating voltage of 75 kV. All chemicals were obtained from Polysciences (Warrington, PA) unless otherwise noted. Parasite acquisition and culture Adult S. mansoni (7 weeks post infection) were obtained from infected mice by hepatic portal vein perfusion [59] with 37 °C DMEM (Mediatech, Manassas, VA) plus 5% fetal calf serum (FBS, Hyclone/Thermo Scientific). Parasites were rinsed several times in DMEM+5% FBS, male and female parasites were separated by incubation (2–3 min) in a 0.25% solution of the anaesthetic ethyl 3-aminobenzoate methanesulfonate (Sigma-Aldrich) in DMEM+5% FBS. Vertebrate animal care In adherence to the Animal Welfare Act and the Public Health Service Policy on Humane Care and Use of Laboratory Animals, all experiments with and care of vertebrate animals were performed in accordance with protocols approved by the Institutional Animal Care and Use Committee (IACUC) of the University of Illinois at Urbana-Champaign (protocol approval number 10035). Accession Codes: Sequence data have been deposited in GenBank/EMBL/DDBJ under accession numbers KC736555 ( dmd-1 splice form 1), KC736556 ( dmd-1 splice form 2), KC736557 ( dmd-1 splice form 3), KC736558 ( dmd-1 splice form 4), KC736559 ( dmd-2 splice form 1), KC736560 ( dmd-2 splice form 2), KC736561 ( dmd-3 ) and KC736562 ( dmd-4 ). How to cite this article: Chong, T. et al . A sex-specific transcription factor controls male identity in a simultaneous hermaphrodite. Nat. Commun. 4:1814 doi: 10.1038/ncomms2811 (2013).